Aridity threshold in controlling ecosystem nitrogen cycling in arid and semi-arid grasslands Higher aridity and more extreme rainfall events in drylands are predicted due to climate change. Yet, it is unclear how changing precipitation regimes may affect nitrogen (N) cycling, especially in areas with extremely high aridity. Here we investigate soil N isotopic values (δ 15 N) along a 3,200 km aridity gradient and reveal a hump-shaped relationship between soil δ 15 N and aridity index (AI) with a threshold at AI=0.32. Variations of foliar δ 15 N, the abundance of nitrification and denitrification genes, and metabolic quotient along the gradient provide further evidence for the existence of this threshold. Data support the hypothesis that the increase of gaseous N loss is higher than the increase of net plant N accumulation with increasing AI below AI=0.32, while the opposite is favoured above this threshold. Our results highlight the importance of N-cycling microbes in extremely dry areas and suggest different controlling factors of N-cycling on either side of the threshold. Arid and semi-arid biomes cover approximately 41% of the global terrestrial area and provide crucial ecosystem services (for example, food, fibre, biofuel and biodiversity) to a fast-growing global population [1] . As a consequence of global warming and associated climate change, the total area of drylands is predicted to increase globally [2] ; more extreme climatic regimes will make arid and semi-arid ecosystems more vulnerable to increased risk of drought as well as increased probability of intense rain [3] , [4] , [5] . Assessing this vulnerability is a major challenge for ecologists and land managers in developing effective adaptation strategies. Biogeochemical cycling of nutrient elements such as nitrogen (N) is at the core of ecosystem functioning, because N, an essential nutrient element, is the most common limiting nutrient for plant growth, maintenance and reproduction in terrestrial ecosystems [6] . Identifying abrupt changes or tipping points in the relationship between aridity and ecosystem N-cycling can reveal critical vulnerabilities of dryland ecosystems to global climate change. Natural abundance of N isotopes (δ 15 N) can provide insights into large-scale N dynamics in terrestrial ecosystems and has become an effective tool for understanding ecosystem N-cycling [7] , [8] . Investigating spatial variability of soil and plant δ 15 N across an aridity gradient affords an opportunity to evaluate changes of water–nitrogen interactions [9] . Soil δ 15 N has been used as an indicator of the ‘openness’ of N-cycling in an ecosystem (the ratio of N loss to internally cycled N), because 14 N is preferentially lost from the ecosystem, causing the enrichment of 15 N in soils in ecosystems with higher degree of openness in N-cycling [10] . N-cycling in dry sites is considered more open than that in wet sites because soil δ 15 N values tend to be negatively correlated with mean annual precipitation (MAP) at the global scale [11] , [12] . However, the mechanisms underlying the disproportionate loss of inorganic N and the higher enrichment of 15 N in dryland soils are still unclear. More critically, there is a dearth of data from arid areas (that is, aridity index (AI)<0.2 or MAP<200 mm) [11] , [12] , where controls of climatic variables on N isotopes remain largely unknown. To address this major gap, we sampled at multiple points along a transect across arid and semi-arid regions in China, 3,200 km in length and covering an aridity gradient from AI=0.03 to AI=0.57 ( Fig. 1 ). We show soil δ 15 N decreases with increasing AI in areas with 0.32<AI<0.57 (a pattern congruent with other studies), but surprisingly increases with increasing AI in areas with AI<0.32, showing a threshold at AI=0.32. Variations of foliar δ 15 N, nitrification and denitrification gene abundance and metabolic quotient for CO 2 (qCO 2 ) along the gradient provide further evidence for the existence of this threshold. These results suggest the importance of N-cycling microbes in extremely dry areas and the different controlling factors and mechanisms of N-cycling on the two sides of the threshold. If future climate change pushes aridity over the threshold, responses of microbes and plants may have profound impacts on nutrient cycling, biodiversity conservation and ecosystem services of arid and semi-arid areas. 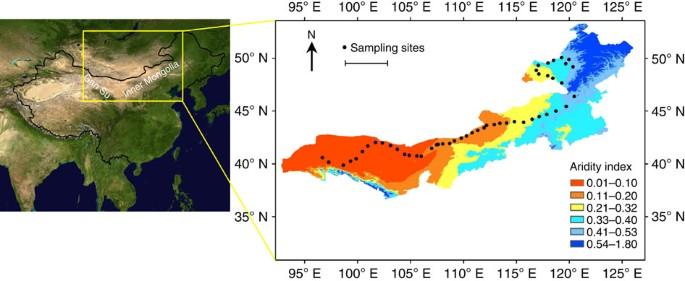Figure 1: Study area and sampling sites. A 3,200 km transect in grasslands of northern China was sampled, from Gansu province to Inner Mongolia. Satellite image is from NASA (National Aeronautics and Space Administration). Aridity index (AI) is the ratio of precipitation to evapotranspiration (data from ref.51), and covers from 0.03 to 0.57. A total of 50 sampling sites were selected (black dots) along this AI gradient. Scale bar, 500 km. Figure 1: Study area and sampling sites. A 3,200 km transect in grasslands of northern China was sampled, from Gansu province to Inner Mongolia. Satellite image is from NASA (National Aeronautics and Space Administration). Aridity index (AI) is the ratio of precipitation to evapotranspiration (data from ref. 51 ), and covers from 0.03 to 0.57. A total of 50 sampling sites were selected (black dots) along this AI gradient. Scale bar, 500 km. Full size image Variations of soil δ 15 N along the transect AI (the ratio of precipitation to potential evapotranspiration) was highly positively correlated with MAP ( r =0.996, Supplementary Table 1 ) and negatively correlated with mean annual temperature (MAT, r =−0.944, Supplementary Table 1 ) along the transect. Therefore, this aridity gradient can also be considered as a MAP gradient or a MAT gradient ( Supplementary Fig. 1 ). Soil δ 15 N did not show a simple linear correlation with AI, instead, showed a hump-shaped one with the maximum at AI=0.32 ( Fig. 2a ). Thus, AI=0.32 was the threshold where water–nitrogen interactions diverged. Our results, to the best of our knowledge, for the first time showed a positive correlation between soil δ 15 N and AI ( Fig. 2a , or between soil δ 15 N and MAP, Supplementary Fig. 2a ) in areas with AI<0.32, which is contrary to the general pattern previously reported [9] , [13] . Soil δ 15 N did exhibit a negative correlation with AI ( Fig. 2a , or between soil δ 15 N and MAP, Supplementary Fig. 2a ) when 0.32<AI<0.57. 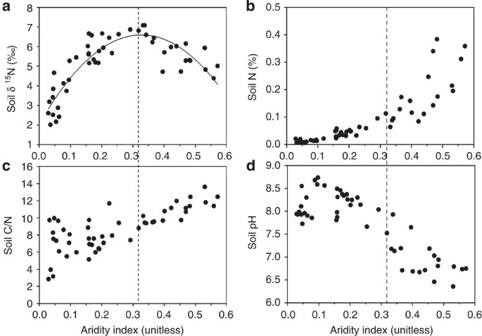Figure 2: Soil N isotopes and edaphic characteristics. Soil δ15N (a), total nitrogen concentration (Soil N,b), soil C/N ratio (c) and pH (d) of study sites along an AI gradient. A second-order polynomial fit well described the relationship between AI and soil δ15N(R2=0.76) and the maximum of this curve was at AI=0.32. Soil N concentration, C/N ratio and pH showed different patterns with increasing AI above and below the threshold AI=0.32. Figure 2: Soil N isotopes and edaphic characteristics. Soil δ 15 N ( a ), total nitrogen concentration (Soil N, b ), soil C/N ratio ( c ) and pH ( d ) of study sites along an AI gradient. A second-order polynomial fit well described the relationship between AI and soil δ 15 N (R 2 =0.76) and the maximum of this curve was at AI=0.32. Soil N concentration, C/N ratio and pH showed different patterns with increasing AI above and below the threshold AI=0.32. Full size image Variations of plant δ 15 N along the transect Foliar δ 15 N of six examined genera generally exhibited a decreasing trend along the AI gradient ( Fig. 3 ), which is consistent with numerous other studies at regional [13] and global [7] , [12] scales. In areas with AI<0.32, foliar δ 15 N of Stipa , Leymus , Reaumuria and Salsola did not correlate with AI, while foliar δ 15 N of Cleistogenes ( y =−8.88 x +3.26, Fig. 3c ) and Caragana ( y =−22.20 x +6.96, Fig. 3d ) correlated negatively with AI. When all genera were lumped, a clear trend was not found in areas with AI<0.32 between foliar δ 15 N and AI, either ( Supplementary Fig. 3a ). In areas with 0.32<AI<0.57, a negative correlation between foliar δ 15 N and AI was observed for Stipa ( y =−15.79 x +8.36, Fig. 3a ) , Leymus ( y =−8.96 x +6.00, Fig. 3b ) and Cleistogenes ( y =−14.36 x +6.22, Fig. 3c ) and there were not enough data points for Caragana ( Fig. 3d ), Reaumuria ( Fig. 3e ), and Salsola ( Fig. 3f ). When all genera were lumped, a negative correlation between AI and foliar δ 15 N was found in areas with 0.32<AI<0.57 ( Supplementary Fig. 3a ). Root δ 15 N was highly correlated with foliar δ 15 N and exhibited similar trend as foliar δ 15 N along the gradient ( Fig. 3 and Supplementary Fig. 3b ). 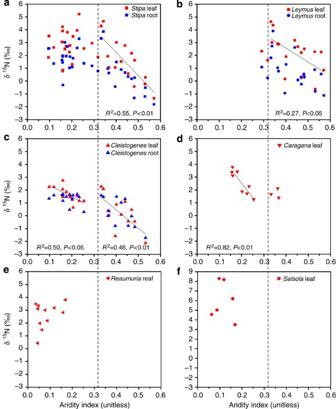Figure 3: Correlation between plant δ15N and AI. Relationship between AI and foliar δ15N (red points) and root δ15N (blue points) of six examined generaStipa(a),Leymus(b),Cleistogenes(c),Caragana(d),Reaumuria(e) andSalsola(f). AI=0.32 was used to separate the data (dashed line) and linear regressions were performed between AI and foliar δ15N at both sides when data points were more than 3. Significant correlations were shown with solid lines. The relationship between root δ15N and AI was similar to that between foliar δ15N and AI, hence was not presented. Figure 3: Correlation between plant δ 15 N and AI. Relationship between AI and foliar δ 15 N (red points) and root δ 15 N (blue points) of six examined genera Stipa ( a ), Leymus ( b ), Cleistogenes ( c ), Caragana ( d ), Reaumuria ( e ) and Salsola ( f ). AI=0.32 was used to separate the data (dashed line) and linear regressions were performed between AI and foliar δ 15 N at both sides when data points were more than 3. Significant correlations were shown with solid lines. The relationship between root δ 15 N and AI was similar to that between foliar δ 15 N and AI, hence was not presented. Full size image Variations of other biotic factors along the transect Soil N content increased slightly with the increase of AI in areas with AI<0.32, and increased greatly with increasing AI in areas with 0.32<AI<0.57 ( Fig. 2b ). Soil C/N ratio did not show any pattern when AI<0.32, but increased with AI when 0.32<AI<0.57 ( Fig. 2c ). Above-ground net primary production (ANPP, y=386.33 x −10.46, Fig. 4a ) and the standardized abundance of nitrification and denitrification genes based on array probes and DNA concentrations in a gram of soil all increased with AI (when AI<0.32, y=223.98 x −11.80 for nitrification gene and y =116.28 x −5.98 for denitrification gene; when 0.32<AI<0.57, no correlation for nitrification genes and y =88.51 x +3.28 for denitrification gene, Fig. 4b ). However, the standardized abundance of nitrification and denitrification genes based on array probes increased first ( y =8.48 x +2.06 and y =3.52 x +1.31 for nitrification and denitrification genes, respectively, AI<0.32) and then decreased ( y =−1.86 x +3.37 and y =−0.64 x +1.82, for nitrification and denitrification genes, respectively, 0.32<AI<0.57) along the AI gradient and showed a tipping point at AI=0.32 ( Fig. 4c ). In addition, metabolic quotient for CO 2 (qCO 2 =soil respiration divided by microbial biomass C) was used as an index of the ecological efficiency use of the soil microbial community [14] , [15] . qCO 2 showed a negative correlation with AI when AI<0.32 ( y =−0.10 x +0.03) and a positive correlation with AI when 0.32<AI<0.57( y =0.06 x −0.01; Fig. 4d ). 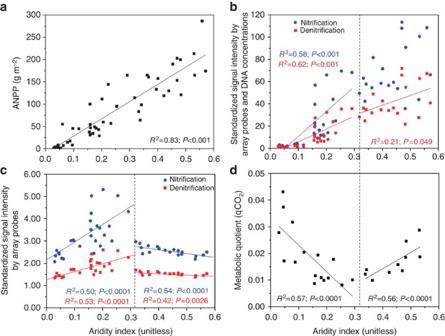Figure 4: Changes of plant and microbial properties with increasing AI. Above-ground net primary production (ANPP) was correlated positively with aridity index (AI;a). Relationships below and above the threshold AI=0.32 were different for the standardized signal intensity based on array probes (c), standardized signal intensity in terms of both array probes and DNA concentrations in a gram of soil (b) and metabolic quotient qCO2(d). Figure 4: Changes of plant and microbial properties with increasing AI. Above-ground net primary production (ANPP) was correlated positively with aridity index (AI; a ). Relationships below and above the threshold AI=0.32 were different for the standardized signal intensity based on array probes ( c ), standardized signal intensity in terms of both array probes and DNA concentrations in a gram of soil ( b ) and metabolic quotient qCO 2 ( d ). Full size image Structural equation model (SEM) showed that AI was the most significant factor influencing ecosystem δ 15 N among AI, soil N, soil clay content, soil pH, soil C/N, ANPP, denitrification gene abundance and N deposition rate ( Supplementary Fig. 4 ). The opposite relationship between soil δ 15 N and AI for below and above AI=0.32 suggests that the controlling factors and mechanisms of N-cycling were different in areas below and above this threshold. Considering soil as a well-mixed ‘black box’, soil δ 15 N is only determined by input and output pathways of 15 N to and from soils [16] . Seven processes affecting soil δ 15 N include ( Supplementary Fig. 5 ): (1) N deposition; (2) N 2 fixation; (3) nitrification and denitrification by microbes which produce gaseous products; (4) NH 3 volatilization; (5) abiotic gaseous N losses; (6) N leaching losses; and (7) net plant N accumulation (plant N uptake minus plant litter N return). δ 15 N of N input by deposition and fixation (processes 1 and 2) is close to zero and is generally lower than soil δ 15 N (ref. 17 ). Therefore, the input processes would reduce soil δ 15 N and if there were no N losses from the soil, soil δ 15 N would be close to δ 15 N of N input (≈0‰). However, the range of our soil δ 15 N was 2–7‰, which means output processes leaving more 15 N in the soil enriched soil 15 N compared with the inputs. The output processes, including gaseous N losses (process 3, 4 and 5), leaching (process 6) and net plant N accumulation (process 7), have different isotope enrichment factors ( Supplementary Fig. 5 ). Gaseous N losses are mainly composed of NH 3 from volatilization and NO, N 2 O and N 2 from nitrification and denitrification, which have the highest isotopic fractionation factor ( ε G ≈16–30‰) [11] , [18] . The isotopic fractionation effect of N leaching losses is the lowest ( ε L ≈1‰) [18] , [19] , while that of net plant N accumulation is in the middle ( ε p ≈5–10‰) [11] , [20] . Hence, soil δ 15 N is determined by the balance of these input and output processes and their enrichment factors. After Brenner et al . [16] and Bai and Houlton [21] , a model can be used to estimate soil δ 15 N: where δ 15 N soil and δ 15 N input are soil and input δ 15 N, respectively; f gas , f leaching and f plant are the fraction of gaseous N losses, N leaching losses and net plant N accumulation out of total losses (%), respectively. Therefore, we get: In extremely dry areas (that is, AI<0.32), N leaching losses are negligible and only gaseous N losses and net plant N accumulation contribute to N losses ( f gas + f plant =1). We can get: Because ε G > ε p , δ 15 N soil is positively correlated with f gas . Therefore, the positive correlation between AI and soil δ 15 N observed in areas with AI<0.32 may be mainly due to increase of f gas . Changes of δ 15 N input , ε G and ε p may also be the potential reasons, however, their variations are within a certain range so that they alone may not be enough to cause such a significant change and correlation [17] , [22] . In fact, we observed higher abundance of nitrification and denitrification genes with increasing AI ( Fig. 4b,c ), which can be considered as an indicator of soil nitrification and denitrification rates [23] , [24] , [25] , and therefore, gaseous N losses. This result is actually consistent with previous modelled effects of rainfall on rates of N-cycling microbial activities [26] . On the other hand, plant N uptake usually increases with rainfall due to the stimulation of higher water availability [27] , [28] . We observed increased ANPP with increasing AI, pointing to potentially higher net plant N accumulation ( Fig. 4a ). To have a higher f gas with the increase of AI, the increase of gaseous losses (NH 3 , NO x , N 2 O and N 2 ) must be higher than the increase of net plant N accumulation. According to Equation (1), the negative relationship between AI and soil δ 15 N in areas with 0.32<AI<0.57 may be mainly due to the following reasons. First, N deposition rate increased along the gradient ( Supplementary Fig. 6 ) while percentage of legume biomass (potentially N 2 -fixing capacity) did not change ( Supplementary Fig. 7 ) and the δ 15 N value of N deposition may be lower than δ 15 N of N 2 fixation [29] , resulting in lower δ 15 N input and thus lower soil δ 15 N. Second, in these drylands, losses through N leaching should be low relative to other loss pathways. Soil δ 15 N is mainly affected by gaseous N losses and net plant N accumulation. With the increase of AI, the negative correlation between AI and soil δ 15 N indicated a decrease of f gas , or an increase of f plant . Because both gaseous N losses (reflected by nitrification and denitrification genes, Fig. 4b ) and net plant N accumulation (reflected by ANPP, Fig. 4a ) increased with increasing AI, in order to have an increase of f plant , the increase of net plant N accumulation must be higher compared with the increase of gaseous losses. This means in areas with 0.32<AI<0.57, ecosystem N retention rate increased with increasing AI. In summary, in areas with AI<0.32, the increase of gaseous N losses was most likely higher than the increase of net plant N accumulation along the gradient, while in areas with 0.32<AI<0.57, the increase of net plant N accumulation was most likely higher than the increase of gaseous N losses, resulting in opposite relationship between AI and soil δ 15 N below and above the threshold. On the basis of the above reasoning, we propose the following two hypotheses for the N-cycling in our studied drylands. First, highly pulsed rainfall events typically found in drylands [30] , [31] may decouple plant N uptake with soil microbial N transformation in areas with AI<0.32. When the threshold AI=0.32 was passed, these two processes are probably coupled, resulting in higher N retention efficiency (that is, higher f plant ) with increasing AI. Soil microbes may be activated by small rainfall events at lower threshold compared with plants [30] , [32] . As microbial mineralization of soil organic matter is typically the main source of soil inorganic N [33] , if soil microbes are activated by rainfall, there may be a pulse of high N availability to plants [4] . But if there is an asynchrony in N-cycling via water limitation on plant N uptake, the mineralized N is subject to nitrification and denitrification losses. We speculated this to be the main reason as to why the increase of gaseous losses was higher than the increase of net plant N accumulation with increasing AI in areas with AI<0.32. Higher soil N 2 O and other NO X losses from arid land compared with mesic areas have been widely observed [9] , [34] . Our plant δ 15 N and soil nitrification and denitrification gene data provided further evidence to this hypothesis. Leaf δ 15 N of most plant genera did not correlate with AI in areas with AI<0.32 ( Fig. 3 ), indicating minor effect of rainfall on plant N status below the threshold. Although AI negatively affected foliar δ 15 N of Cleistogenes when AI<0.32, its effect was much smaller (slope=−8.88, Fig. 3c ) compared with when AI>0.32 (slope=−14.36, Fig. 3c ). N 2 -fixing genus Caragana was different from other genera, in that its leaf δ 15 N correlated negatively with AI when AI<0.32. This is probably because nitrogenase is significantly affected by water availability and temperature [35] . The standardized abundance of denitrification gene in soil (or nitrification gene), based on array probes and DNA concentrations in a gram of dry soil, increased faster with increasing AI below the threshold ( R 2 =0.62, slope=116.28) than above the threshold ( R 2 =0.21, slope=88.51; Fig. 4b ). The standardized abundance of nitrification and denitrification genes based on array probes also showed the hump-shaped relationship with AI ( Fig. 4c ), indicating the highest importance of N-cycling microbes at the threshold AI=0.32. In addition, qCO 2 was lowest at AI=0.32 ( Fig. 4d ), showing highest carbon use efficiency and ecosystem successional stability at AI=0.32. A previous study in the same area suggested that principal component 1 of phospholipid fatty acid as an indicator of soil microbial community structure showed a hump-shaped relationship along a MAP gradient with the tipping point at approximately AI=0.30 (ref. 36 ). These results together suggest that in extremely dry areas (that is, AI<0.32), although severely constrained by abiotic factors, soil microbes have a very important role in N-cycling and ecosystem function and this importance increases with increasing AI. When the threshold is passed, microbes are less influenced by aridity and plants respond more to aridity variation. Alternatively, abiotic processes such as solar radiation-stimulated N losses may overpower biotic processes in their controls on N-cycling [37] when AI<0.32. ANPP and abundance of nitrification and denitrification genes were low in extremely dry areas, especially when AI<0.10 ( Fig. 4a,b ); thus abiotic processes may be major contributors to gaseous N losses. Ammonia volatilization, which has a high isotope fractionation factor [11] , can be a key abiotic process responsible for gaseous N loss in extremely dry areas where soil pH, a main driver for ammonia volatilization, tended to be high ( Fig. 2d ). Abiotic losses of oxidized gaseous N have also been found previously in deserts with MAP=140 mm (ref. 38 ). The opposite relationship between AI and soil δ 15 N over the threshold highlights the need to understand abiotic N-cycling in those extremely dry areas. If future climate change leads to higher aridity in dry areas [2] , once the AI threshold is passed, N-cycling in dry ecosystems may diverge due to the nonlinearity of the controlling mechanism of water–nitrogen interactions and plant–microbe interactions. For example, plants currently existing in areas with AI>0.32 are adapted to pulsed rainfall stimulation of N uptake [39] , and once the aridity is increased these plants may be more N limited and even become extinct. On the other hand, because plants in areas with AI<0.32 are adapted to the extremely dry condition, future longer dry cycle [4] may affect soil microbes more than plants in those areas. More importantly, the uncoupled plant and microbial response to pulsed rainfall events in areas with AI<0.32 makes arid ecosystem highly vulnerable to future climate change. The relationship between AI and soil δ 15 N revealed in this study suggests that the pattern of N-cycling along the AI gradient in arid and semi-arid ecosystems is nonlinear with a threshold value of approximately AI=0.32. This new nonlinear relationship stresses the need to incorporate the nonlinearity between aridity and N-cycling into process-based models for better predicting possible responses of drylands to future climate change. For example, denitrifiers (or nitrifiers) should respond to aridity or rainfall in extremely dry areas differently from that of low-aridity areas. Microbial N pools and processes should be given more weightage than plant pools when modelling N cycling in extremely dry areas. The stimulation of pulse rainfall events to microbes and plant N uptake should be modelled differently, with a lower stimulation threshold for microbes in extremely dry areas [32] . The generality of our findings warrants further research in other arid and semi-arid regions. Overall, our findings highlight the importance of changing precipitation regimes on nutrient cycling, biodiversity conservation and ecosystem services of arid and semi-arid areas. Sampling sites This study was conducted along a 3,200-km west–east transect across Gansu province and Inner Mongolia in northern China ( Fig. 1 ). Longitude of the transect covered approximately 24° ranging from 96°40′ to 120°28′ and latitude ranged from 39°51′ to 50°30′. The climate was predominantly arid and semi-arid continental; MAP ranged from 34 to 436 mm and mean annual air temperature (MAT) ranged from −5 to 10 °C.The main vegetation types that distributed from the west to east across this transect were desert steppe, typical steppe and meadow steppe. Soil types were predominantly arid, sandy, brown loess rich in calcium, and belonged to Kastanozem soil group in the Food and Agriculture Organization (FAO) classification system [40] . In the 2012 field campaign, we selected 50 sites through the entire transect ( Fig. 1 ). Most of the sampling sites were far from cities and were considered as under natural conditions without significant human influences ( Supplementary Fig. 8 ). At each site, two 50 m × 50 m large plots were established and five 1 m × 1 m subplots (or five 5 m × 5 m subplots in areas dominated by shrubs) were selected within each large plot (each corner and the centre of the plot). The spatial geographical coordinates and elevation of each site were recorded by GPS (eTrex Venture, Garmin, USA). In each 1 m × 1 m subplot, after harvesting all grasses for calculation of ANPP, twenty random soil samples (0–10 cm) were collected using a soil corer (2.5-cm diameter), and were mixed thoroughly and pooled as one composite sample for subsequent chemical and microbial analysis. In the 5 m × 5 m subplot for shrub sampling, one fourth annual branches of each shrub were clipped for ANPP and then twenty random soil samples (0–10 cm) were collected under shrubs and bare ground and mixed together into one sample. Soil samples were sieved through a 2.0-mm sieve and then separated into two parts: one was stored into a plastic bag in a refrigerator at −4 °C for isotope and incubation experiments; the other one was stored into a sterile plastic bag in a refrigerator at −40 °C for DNA extraction. For plant samples, three dominant grass genera and three shrub genera were selected for isotope analyses: Stipa , Leymus , Cleistogenes , Caragana , Reaumuria and Salsola . For Stipa , Leymus and Cleistogenes , we sampled both leaves and roots. Under the target plant, roots were excavated by extracting a soil cylinder (25 cm in diameter and 30 cm in depth) with the plant in the middle using a spade. The size of the soil cylinder depended on the above-ground morphology of the target plant. After removing the soil, the whole plant was carefully separated into below-ground and above-ground parts by scissors and stored in an envelope, separately. For Caragana , Reaumuria and Salsola , only leaves were sampled. Ten replicates were bulked into a single sample. Leaves showing damage or discolouration were discarded. Plant leaf and root samples were washed with deionized water to remove dust particles and then dried at 65 °C for 48 h for further analyses. Analysis of N isotopes and concentration Soil subsamples were sieved through a 2.0-mm sieve and dried at 65 °C. Both plant and soil samples were ground in a ball mill and then stored in a plastic bag until further analysis. Following the method described by Harris et al . [41] , all soil samples were washed using 150 ml of 0.5 M HCl to remove carbonate before soil organic carbon (SOC) analysis. Another balled soil subsample without HCl treatment was used to analyse total N concentration and N isotope ratios. All analyses for SOC, total N concentration and N isotope ratios were carried out at the Stable Isotope Faculty of University of California, Davis. About 3 mg of leaf and root samples and 65 mg of soil samples were loaded into a capsule and determined using an Elementar Vario EL Cube (Elementar Analysis system GmbH, Hanau, Germany) interfaced to a PDZ Europa 20-20 isotope ratio mass spectrometer (Sercon Ltd., Cheshire, UK), with an overall precision better than 0.2‰. Isotope value was expressed in parts per thousand (‰) relative to air N 2 for 15 N/ 14 N, using standard delta (δ) notion. Analysis of soil properties We measured soil microbial biomass carbon (C) using the chloroform fumigation–extraction method [42] . Briefly, one subsample (10 g) sieved through 2.0 mm was extracted with 0.5 M K 2 SO 4 solution for 2 h on an end-over-end shaker, and another subsample (10 g) was fumigated by ethanol-free chloroform in the dark for 48 h and then extracted with 0.5 M K 2 SO 4 solution for 2 h on an end-over-end shaker. The concentration of total organic C in each extract was analysed by the total organic carbon analyser. The difference between C extracted from fumigated and non-fumigated samples was converted into C in the microbial biomass by using a coefficient 2.64 (ref. 43 ). A subsample soil (10 g) sieved through a 2.0 mm sieve was used for pH value in water at a 1:2.5 soil/water ratio and another subsample was fractionated into sand (particle size, 50–300 μm), silt (2–50 μm) and clay (<2 μm) using ultrasonic energy method [44] . All results of particle size analysis were expressed as the percentage, by weight, of the oven-dried soil. Soil basal respiration was determined using incubation method in laboratory. Soil samples were incubated for 6–48 h depending on SOC concentration with soil moisture at 60% of field capacity at 25 °C. Twenty-six sites were selected from the total 50 sampling sites, with every other site from west to east along the transect being selected. Then 150 g air-dried soil of each site (three replicates) was put into a 1,000-ml wide-mouth glass bottle covered with a piece of parafilm (Parafilm M, Bemis, USA) that is moisture-resistant but allows aeration. The bottle was placed in an incubator (SPX-250B5H, CIMO, China) at 25 °C for 15 days for pre-incubation so that microbes could get used to the environment, and soil respiration was relatively stable. Following the pre-incubation, we used a rubber septa, which had a long inlet tube and a short outlet tube, to seal the wide-mouth bottle. CO 2 -free air was blown through the long inlet tube for half an hour to remove residual CO 2 in the bottle. We then closed both inlet and outlet tubes and incubated the soil for 6–48 h depending on soil C concentration. After the incubation, headspace CO 2 in the bottle was pumped out through the short outlet tube using a gas-tight syringe (Monoject, Tyco Healthcare, USA) and injected into Los Gatos Research Carbon Dioxide Isotope Analyser (LGR-CCIA-36d, LGR, USA) to measure CO 2 concentration (p.p.m.). Soil basal respiration was assumed to be equal to the increase in CO 2 concentration over the incubation period. The metabolic quotient for CO 2 (qCO 2 ) was calculated as the ratio of basal respiration to microbial biomass C 14 . High qCO 2 means inefficient use of energy (high maintenance carbon) or successionally unstable ecosystems and low qCO 2 means high energy use efficiency and stable ecosystems [45] . DNA extraction and GeoChip analysis Soil DNA was extracted from each of the collected soil samples using the MoBioPowerSoil DNA isolation kit (MoBio Laboratories, Carlsbad, CA, USA) according to the manufacturer’s protocol. For the samples with low biomass, the soil DNAs were extracted using the method of freeze-grinding and SDS-based lysis as described previously [46] . The quality of the purified DNAs was assessed on the basis of the ratios of 260/280 nm and 260/230 nm absorbance by a NanoDrop ND-1000 Spectrophotometer (NanoDrop Technologies Inc., Wilmington, DE). The final DNA concentrations were quantified by PicoGreen [47] using a FLUOstar Optima (BMG Labtech, Jena, Germany). The latest generation of functional gene array, GeoChip 5.0S, was used to analyse the functional structure of the soil microbial communities. The GeoChip 5.0S contained more than 57,000 oligonucleotide probes, covering over 144,000 gene sequences from 393 gene families. Nineteen main functional gene groups are involved in N cycling, such as nitrification (amoA, hao), denitrification (narG, nirK, nirS, norB, nosZ), nitrogen fixation (nifH) and so on. GeoChip 5.0S was manufactured by Agilent (Agilent Technologies Inc., Santa Clara, CA) in the 8 × 60 K format. The purified soil DNAs (0.6 μg) was used for GeoChip 5.0S hybridization, which was labelled with Cy 3 as described previously [48] , [49] , [50] . Before hybridization, the labelled DNA was re-suspended and hybridized with GeoChip 5.0S. The hybridization solution (42 μl in total) contained 1 × HI-RPM hybridization buffer, 1 × Acgh blocking, 0.05 μg/μl Cot-1 DNA, 10 pM universal standard DNA and 10% formamide (final concentrations). GeoChip hybridization was carried out at 67 °C in Agilent hybridization oven for 24 h. After hybridization, the slides were washed with Agilent Wash Buffers at room temperature. The arrays were then scanned with a NimbleGen MS200 Microarray Scanner (Roche NimbleGen, Inc., Madison, WI, USA) at 633 nm using a laser power of 100% and a photomultiplier tube gain of 75%. The images data were extracted by Agilent Feature Extraction program. The microarray data were preprocessed for subsequent analysis as described previously [48] , [49] , [50] in terms of poor and outlying spot removal, background subtraction, normalization and sample. Data sources AI (the ratio of precipitation to potential evapotranspiration), MAP and MAT of each sampling site were calculated from the WorldClimdatabase [51] . N deposition rate ( Supplementary Fig. 6 ) of each site was estimated using the data of Lelieveld and Dentener [52] and the distance of each sampling sites to the nearest city was calculated using Google Map ( Supplementary Fig. 7 ). All data extraction was processed in ArcGIS version 9.3 using Spatial Analysis tool (ESRI, Redlands, CA). Data analyses We explored the relationship of AI with the soil δ 15 N and found that the relationship was well described by a second-order polynomial fit, with the maximum of the curve at AI=0.32. Therefore, AI=0.32 was used as the threshold for all regression analyses. Ordinary least squares regression analysis was conducted to examine all the linear relationships between AI and soil characteristics. Differences in slopes of ordinary least squares regressions were tested by one-way analysis of covariance using SPSS 18.0 (SPSS, Chicago, IL) for windows. GeoChip contains probes from various gene categories, but their total signal intensity of the detected probes could not be used directly to estimate the relative differences of individual gene categories across different samples because the total numbers of probes on the arrays vary substantially among different gene categories [51] . Thus, the signal intensity detected under each gene category was standardized by dividing the total signal intensity of the detected probes in a gene category (for example, nitrification, denitrification) with the total number of the probes of that category on the array as presented in Fig. 4c . In addition, the standardized signal intensity was further expressed in a gram of dry soil based on DNA quantity as presented in Fig. 4b . To address how AI, edaphic variables (pH, soil N concentration, soil C/N ratio and soil clay content), ANPP, N deposition and denitrification gene abundance interactively affected soil and plant δ 15 N, SEM was applied ( Supplementary Fig. 4 ). We started the SEM procedure with the specification of a conceptual model of hypothetical relationships, based on a priori and theoretical knowledge. In the SEM analysis, we compared the model-implied variance–covariance matrix against the observed variance–covariance matrix. Data were fitted to the models using the maximum-likelihood estimation method. For simplicity, the least significant path was deleted and the model was re-estimated; then the next least significant path was removed, and so on, until the paths that remained in the final SEM was all significant. Nonsignificant χ 2 tests ( P >0.05) and CFI (comparative fit index) values >0.90 were considered acceptable [53] . How to cite this article: Wang, C. et al . Aridity threshold in controlling ecosystem nitrogen cycling in arid and semi-arid grasslands. Nat. Commun. 5:4799 doi: 10.1038/ncomms5799 (2014). Accession codes: Microarray data have been deposited in the ArrayExpress database under accession code E-MTAB-2722 .